Observation of coherent quench dynamics in a metallic many-body state of fermionic atoms Quantum simulation with ultracold atoms has become a powerful technique to gain insight into interacting many-body systems. In particular, the possibility to study nonequilibrium dynamics offers a unique pathway to understand correlations and excitations in strongly interacting quantum matter. So far, coherent nonequilibrium dynamics has exclusively been observed in ultracold many-body systems of bosonic atoms. Here we report on the observation of coherent quench dynamics of fermionic atoms. A metallic state of ultracold spin-polarized fermions is prepared along with a Bose–Einstein condensate in a shallow three-dimensional optical lattice. After a quench that suppresses tunnelling between lattice sites for both the fermions and the bosons, we observe long-lived coherent oscillations in the fermionic momentum distribution, with a period that is determined solely by the Fermi–Bose interaction energy. Our results show that coherent quench dynamics can serve as a sensitive probe for correlations in delocalized fermionic quantum states and for quantum metrology. The investigation of nonequilibrium dynamics in interacting quantum many-body systems has emerged as a major research direction in the field of ultracold atoms. It provides unique insight into quantum states, their excitation spectra [1] , [2] , [3] and thermalization processes [4] , [5] . Time evolution far from equilibrium has primarily been studied using purely bosonic systems, allowing the observation of coherent quench dynamics [6] , [7] , [8] , [9] and equilibration [10] , [11] , [12] in isolated setups. Close to equilibrium, various driving protocols have been devised to use dynamics as a means for obtaining information about the excitation spectra of many-body phases in optical lattices [13] , [14] , [15] , [16] . Centre of mass oscillations in a mixture of fermionic and bosonic superfluids have been used to measure the coupling between the two superfluids [17] . In purely fermionic systems, nonequilibrium dynamics has been explored in transport measurements that allowed for a semi-classical theoretical description [18] . However, so far, the observation of coherent nonequilibrium quantum dynamics for fermions has remained elusive. At ultracold temperatures, quantum statistics dominates and gives rise to distinctive many-body ground states for bosonic and fermionic systems [19] . Noninteracting bosons collectively condense into the single-particle state of lowest energy, forming a Bose–Einstein condensate (BEC). Fermions, on the other hand, obey the Pauli exclusion principle, which limits the occupation of single-particle states to a maximum of one fermion. Therefore, fermions fill the lowest energy single-particle states from bottom up and form a Fermi sea. When placed in a periodic lattice potential with M sites, the wavefunction of the BEC can be written as the product [20] of identical coherent states , where | α | 2 is the mean occupation per lattice site and the bosonic creation operator at site j . On the other hand, the wavefunction of an ideal Fermi gas of N identical fermions can be expressed by the product of the N quasi-momentum eigenstates with energy eigenvalues E k smaller than the Fermi energy E F . Here, denotes the fermionic creation operator and r j the position of site j . As long as the fermions do not completely fill up a lattice band, represents a metallic state. The distinct ground state properties of bosons and fermions have direct implications for their respective many-body quantum dynamics. For the case of bosons, coherent quench dynamics was experimentally studied by preparing an atomic BEC in a shallow optical lattice and taking it out of equilibrium by a sudden quench to a deep lattice [6] , [7] , [8] . The rapid suppression of tunnelling and the enhanced interactions between the atoms gave rise to characteristic collapses and revivals of the bosonic matter wave interference pattern, whose periodicity is determined by the strength of the on-site interaction U BB . In homogeneous lattice potentials, this phenomenon can be understood from the dynamics of a single lattice site: The time evolution of the many-body state is governed by the operator with being the on-site interaction term of the Bose–Hubbard Hamiltonian, where counts the number of bosons at site j . Consequently, the dynamics of the entire system, , comprises a product of identical dynamics at each lattice site. In this work, we are concerned with the dynamics of a delocalized many-body state of fermions for which, even in a homogeneous lattice, an effective single-site description is not possible. Specifically, we consider a shallow optical lattice that is simultaneously loaded with a metallic state of spin-polarized fermionic atoms and an atomic BEC, as schematically shown in Fig. 1a . Initially, the interactions between fermions and bosons are weak, while the large kinetic energy dominates. Therefore, we approximate the quantum state of this hybrid Fermi–Bose system by the direct product . When the system is quenched by a rapid increase of lattice depth, tunnelling between lattice sites is suppressed both for fermions and bosons, and interparticle interactions dominate. Interactions among the bosonic component give rise to typical collapse and revival dynamics that has been analysed previously [21] . It is the key finding of the present work that the fermionic component also undergoes coherent dynamics. Although the fermions do not interact among themselves, their interaction with the bosons drives the dynamics of the quenched metallic state. Similar to the purely bosonic case, the time evolution operator factorizes into with being the on-site interaction term of the Fermi–Bose–Hubbard Hamiltonian [22] , where counts the number of fermions at site j and U FB is the on-site Fermi–Bose interaction energy. However, due to its delocalized nature, the initial metallic state does not factorize into a product of on-site wavefunctions. This is crucial for coherent fermionic dynamics to occur, the time scale of which is given by h / U BF . We discuss the role of fermionic and bosonic number fluctuations in the quench dynamics and introduce the visibility of the fermionic momentum distribution as a suitable observable. In the experiment, we study the dynamics for various strengths of the Fermi–Bose interaction and reveal their spectral properties through Fourier analyses. As a result of fermionic quantum statistics, the spectra exclusively reveal the Fermi–Bose interaction energy U FB with high resolution. Coherent quench dynamics can therefore be used as a sensitive probe for correlations and complex interaction effects in hybrid many-body quantum systems. 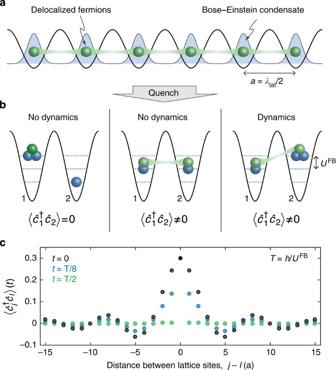Figure 1: Emergence of coherent quench dynamics in a metallic many-body state. (a) A Fermi–Bose quantum gas mixture is loaded into a shallow optical lattice. The spin-polarized fermions form a metallic many-body quantum state, delocalized across the lattice (green spheres). The bosons form a BEC (blue background). (b) A rapid increase of lattice depth quenches the system. The on-site interactions between fermions and bosons,UFB, drive coherent dynamics in the fermionic momentum distribution. The origin of the dynamics is illustrated by considering three sample cases in a two-site system. If the system features a localized fermion (left) or bosonic Fock states with an equal number of bosons on each site (middle), no dynamics occurs. Dynamics occurs if the fermion is delocalized,, and the number of bosons is different on each site (right). (c) Fermionic single-particle correlations in a 1D lattice at timest=0,h/(8UFB) andh/(2UFB) after the quench. The fermionic filling is chosen to beand stays constant as a function of time (black point atj−l=0). Figure 1: Emergence of coherent quench dynamics in a metallic many-body state. ( a ) A Fermi–Bose quantum gas mixture is loaded into a shallow optical lattice. The spin-polarized fermions form a metallic many-body quantum state, delocalized across the lattice (green spheres). The bosons form a BEC (blue background). ( b ) A rapid increase of lattice depth quenches the system. The on-site interactions between fermions and bosons, U FB , drive coherent dynamics in the fermionic momentum distribution. The origin of the dynamics is illustrated by considering three sample cases in a two-site system. If the system features a localized fermion (left) or bosonic Fock states with an equal number of bosons on each site (middle), no dynamics occurs. Dynamics occurs if the fermion is delocalized, , and the number of bosons is different on each site (right). ( c ) Fermionic single-particle correlations in a 1D lattice at times t =0, h /(8 U FB ) and h /(2 U FB ) after the quench. The fermionic filling is chosen to be and stays constant as a function of time (black point at j − l =0). Full size image Quench dynamics in a two-site system To illustrate the emergence of coherent quench dynamics, we consider an elementary setup with two lattice sites [23] (labeled 1 and 2, spaced by distance a ), occupied by a single fermion and multiple bosons (see Fig. 1b ). For finite tunnelling and vanishing interactions, U FB =0, the fermionic ground state has the form , corresponding to the fermion being in the k =0 quasi-momentum eigenstate. After a quench in which interactions between fermions and bosons are turned on and tunnelling amplitudes for fermions and bosons are set to zero, the site occupations remain constant due to the absence of tunnelling. The off-diagonal correlations of the single-particle density matrix, however, evolve in time: , where n 1 ( n 2 ) is the number of bosons on site 1 (2). Consequently, the fermionic quasi-momentum distribution, , undergoes dynamics. The evolution for the two allowed quasi-momentum eigenstates k =0 and k = π / a reads (1±cos[ U FB ( n 1 − n 2 ) t / ℏ ])/2, and indicates that the fermion oscillates between the k =0 and k = π / a states with a period T ∝ h / U FB . In contrast, no dynamics occurs if the fermion initially occupies a localized state, or , as the off-diagonal correlations vanish, or if the number of bosons is identical on both the sites ( n 1 = n 2 ). For n ( k ) to evolve with time, delocalized fermions and spatially varying bosonic occupancies are required. In the experiment, the latter is provided by the quantum fluctuations of the on-site occupation that are characteristic for a BEC. As this specific example of a two-site model only contains one fermion, quantum statistics does not play a role in the dynamics of n ( k ). However, quantum statistics plays an essential role in the dynamics of the quasi-momentum distribution when, as in the experiments, many fermions are present. Fermionic quench dynamics in a lattice system To characterize the quench dynamics in a setup with many lattice sites, it is convenient to study the visibility of the fermionic quasi-momentum distribution. We define it as the ratio between the number of fermions with quasi-momenta in the interval [− k 0 , k 0 ] (see Fig. 2a ) and the total fermion number N , . For the case of a one-dimensional (1D) lattice and an initial state , the time evolution of the visibility after the quench can be calculated analytically in the thermodynamic limit (see Methods). 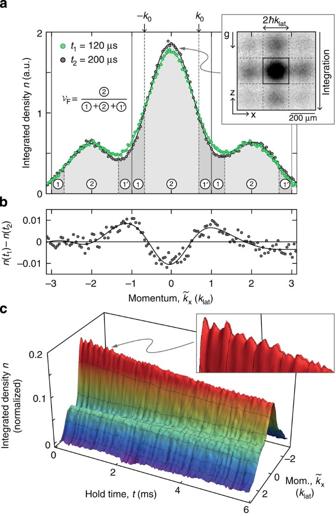Figure 2: Quench dynamics in the momentum distribution of fermionic40K atoms. (a) After variable hold timest, the fermionic momentum distributions are recorded after time-of-flight expansion (inset). Integration along thez-direction results in 1D momentum profiles and averages the effect of Bloch oscillations, which occurs as a consequence of gravity. We show profiles at an interspecies scattering length ofaFB=−161.2(1)a0fort1=120 μs (green) andt2=200 μs (black). Solid lines show a fit of three Gaussians that are separated by the Brillouin zone width 2klat. (b) The residual profileillustrates the redistribution of population within the Brillouin zone. (c) Evolution of the fermionic momentum distribution after the quench. The integrated profiles for each timet,, are normalized to a total area of one. Coherent quench dynamics is visible as a periodic modulation of the peak height at(magnified in the inset). Assuming k 0 ≤ k F , we obtain Figure 2: Quench dynamics in the momentum distribution of fermionic 40 K atoms. ( a ) After variable hold times t , the fermionic momentum distributions are recorded after time-of-flight expansion (inset). Integration along the z -direction results in 1D momentum profiles and averages the effect of Bloch oscillations, which occurs as a consequence of gravity. We show profiles at an interspecies scattering length of a FB =−161.2(1) a 0 for t 1 =120 μs (green) and t 2 =200 μs (black). Solid lines show a fit of three Gaussians that are separated by the Brillouin zone width 2 k lat . ( b ) The residual profile illustrates the redistribution of population within the Brillouin zone. ( c ) Evolution of the fermionic momentum distribution after the quench. The integrated profiles for each time t , , are normalized to a total area of one. Coherent quench dynamics is visible as a periodic modulation of the peak height at (magnified in the inset). Full size image where k F is the Fermi quasi-momentum, k lat = π / a is the quasi-momentum corresponding to the edge of the Brillouin zone and a is the lattice spacing. Analogous to the two-site case, the periodicity of the oscillation is determined by T = h / U FB , and the coherent dynamics originates from the presence of off-diagonal single-particle correlations and on-site occupancy fluctuations of the BEC. Figure 1c illustrates the time evolution of the off-diagonal correlations , where is the fermionic filling. The theoretical analysis can be extended to three-dimensional (3D) lattices, where n ( k x , t ) is taken to be the projection of the full fermionic quasi-momentum distribution n ( k x , k y , k z , t ) onto 1D, . The results are qualitatively similar to equation (1) (see Methods). Experimental sequence and observation of quench dynamics The experiment begins with the preparation of a quantum degenerate mixture of 2.1(4) × 10 5 fermionic 40 K and 1.7(3) × 10 5 bosonic 87 Rb atoms in their absolute hyperfine ground states |9/2, −9/2〉 and |1, +1〉, respectively. The temperature of the spin-polarized Fermi gas is typically T / T F =0.20(2). Its interaction with the bosons is tuned by means of a Feshbach resonance at 546.75(6) G (ref. 24 ), addressing interspecies scattering lengths a FB in a range between −161.2(1) a 0 and +59(10) a 0 . Subsequently, a 3D optical lattice operating at a wavelength of λ lat =738 nm is adiabatically ramped up within 50 ms to a depth of , where denotes the recoil energy, m F the atomic mass of 40 K and k lat =2 π / λ lat (for the corresponding lattice depths for 87 Rb, see Methods). For these parameters, the fermions form a metallic many-body state within the first lattice band (see Methods) [25] and the bosons form a BEC. Then, we quench the system by rapidly increasing the lattice depth to , suppressing the tunnel coupling between the lattice sites and initiating coherent nonequilibrium dynamics of the Fermi–Bose many-body state. After letting the system evolve for variable hold times t , all trapping potentials are suddenly switched off and an absorption image of the momentum distribution of 40 K is recorded after 9 ms time-of-flight expansion (see Fig. 2a , inset). The dynamics of the fermionic many-body state is revealed via oscillations in the momentum distribution (see Fig. 2 ). The recorded absorption images are integrated along the direction of gravity to obtain 1D momentum profiles at discrete hold times t , sampled in steps of 40 μs. Figure 2a compares two such profiles that are recorded at the approximate times of a half and a full oscillation cycle for a fixed value of Fermi–Bose interactions. The residual after subtracting the two profiles one from another (see Fig. 2b ) illustrates how the interaction-driven dynamics leads to a redistribution of the population from the momenta at the centre to the momenta at the edge of the Brillouin zone. The coherent quench dynamics can be observed as a periodic modulation of the peak height at for hold times shorter than the time scale set by residual tunnelling of the fermions. For longer times, the momentum profiles relax towards a state with a more uniform distribution across the Brillouin zone ( Fig. 2c ), as a consequence of equilibration due to residual tunnelling (see Methods). Fermionic visibility A quantitative understanding of the coherent fermionic dynamics can be gained from the time traces of the visibility . For each momentum profile , the fermionic visibility is calculated after adding the regions with momenta (− k lat , −3 k lat ) and ( k lat , 3 k lat ) to the first Brillouin zone (− k lat , k lat ), as illustrated in Fig. 2a . To obtain the largest amplitude of the visibility oscillations, we choose k 0 =2 k lat /3, which is approximately the k -value where the residual profile in Fig. 2b changes sign. 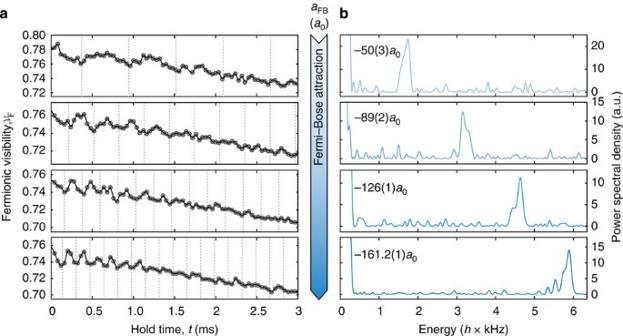Figure 3: Coherent quench dynamics of a metallic many-body state. (a) Time traces of the visibility show the quantum dynamics of fermionic40K atoms, driven by variable attractive interactions with bosonic87Rb atoms. Dashed vertical lines indicate the periodicity of the dynamics. The solid lines interpolate the data and serve as a guide to the eye. Each data point corresponds to a single run of the experiment. (b) Fourier analysis reveals the spectral content of the time traces in (a). Figure 3a shows time traces of the evolution with up to 10 observable oscillation periods. On increasing the attraction between fermions and bosons, the period of the oscillations becomes shorter as expected from the theoretical analysis. This confirms that the quench dynamics is driven by the interspecies interaction U FB ∝ a FB . In general, we observe oscillation amplitudes that are significantly smaller than in the case of bosonic collapse and revival dynamics [6] , [8] . The reason is that only correlations between fermions on sites with bosons contribute to the dynamics, while unaccompanied fermions form a static background. The Fermi–Bose overlap volume is fundamentally limited because the in-trap size of a Fermi gas is significantly larger than a BEC with comparable atom numbers due to Pauli pressure. In addition, differential gravitational sag can lead to a vertical displacement of the two atom clouds. In our setup, those two effects result in about 5% of the fermions overlapping with bosons. This is compatible with the measured oscillation amplitudes (see Methods). Furthermore, finite temperature and Fermi–Bose interactions in the initial state localize fermions [26] , [27] and reduce the visibility. Finally, residual tunnelling after the quench is expected to induce damping and to reduce the oscillation amplitude [28] , [29] . Figure 3: Coherent quench dynamics of a metallic many-body state. ( a ) Time traces of the visibility show the quantum dynamics of fermionic 40 K atoms, driven by variable attractive interactions with bosonic 87 Rb atoms. Dashed vertical lines indicate the periodicity of the dynamics. The solid lines interpolate the data and serve as a guide to the eye. Each data point corresponds to a single run of the experiment. ( b ) Fourier analysis reveals the spectral content of the time traces in ( a ). Full size image The spectral content of the fermionic quench dynamics is revealed via Fourier transform of the visibility time traces (see Methods). As shown in Fig. 3b , the spectra are dominated by a single peak, in remarkable contrast to the complex spectra of the bosonic collapse and revival dynamics in the same experimental setting [21] . Its width of about 300 Hz is compatible with dephasing as a result of both residual tunnelling and a small harmonic anticonfinement (see Methods). The peak also displays a comb-like substructure with several frequencies of order U FB / h . We assign this substructure to the deformation of on-site orbitals as a result of interactions [8] , [27] , [30] that effectively gives rise to an explicit dependence of the Fermi–Bose interaction energy on the bosonic on-site occupation n , (see Methods). According to equation (1), additional peaks at frequencies 2 U FB , 3 U FB , … are expected, but not observed in the spectra. As follows from our discussion of the two-site system, such higher frequency components result from correlations between fermions in lattice sites whose occupations differ by two or more bosons. However, due to the different sizes of the fermion and boson clouds, as well as their differential gravitational sag (see Methods, Supplementary Fig. 1 and Supplementary Note 1 ), such correlations are strongly suppressed in our setup. This results in the suppression of higher harmonics of U FB below the noise level of our spectra. In Fig. 4 , we show the progression of U FB as a function of the interspecies scattering length both for attractive and repulsive Fermi–Bose interactions. We compare the experimental results with the numerical calculations of U FB that use Wannier functions as on-site orbitals. The agreement is remarkable. On the attractive side, the results of the calculations are compatible with the highest frequency components measured experimentally. On the repulsive side, all frequency components measured in the experiments are contained within the bounds of the calculations. 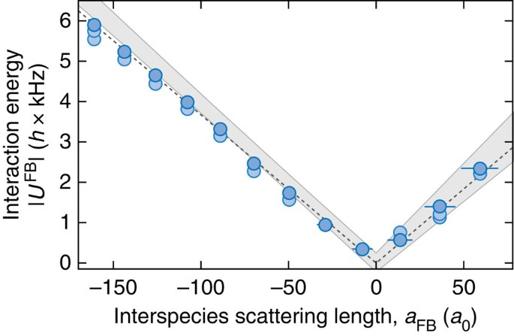Figure 4: Precision measurement of the Fermi–Bose interaction energyUFB. For each interspecies scattering lengthaFBthe dominant spectral components (dark points) and the spectral substructure (light points) are shown. Horizontal error bars reflect the experimental uncertainty (s.d.) of the scattering lengthaFB, vertical error bars are smaller than the size of the data points. The dashed line shows a linear fitC|aFB| to the dominant spectral features, yieldingC=36.7(3) Hz/a0. The shaded area shows a numerical calculation assuming the prescriptionUFB=(2πℏ2aFB/μ)∫dr3|wB(r)|2|wF(r)|2of a single-band Hubbard model, taking into account the experimental uncertainties in lattice depth and interspecies scattering lengthaFB. Here,wF(r) andwB(r) denote the fermionic and bosonic Wannier functions, respectively, andμ=mFmB/(mF+mB) is the reduced mass. Figure 4: Precision measurement of the Fermi–Bose interaction energy U FB . For each interspecies scattering length a FB the dominant spectral components (dark points) and the spectral substructure (light points) are shown. Horizontal error bars reflect the experimental uncertainty (s.d.) of the scattering length a FB , vertical error bars are smaller than the size of the data points. The dashed line shows a linear fit C | a FB | to the dominant spectral features, yielding C =36.7(3) Hz/ a 0 . The shaded area shows a numerical calculation assuming the prescription U FB =(2 π ℏ 2 a FB / μ )∫ dr 3 | w B ( r )| 2 | w F ( r )| 2 of a single-band Hubbard model, taking into account the experimental uncertainties in lattice depth and interspecies scattering length a FB . Here, w F ( r ) and w B ( r ) denote the fermionic and bosonic Wannier functions, respectively, and μ = m F m B /( m F + m B ) is the reduced mass. Full size image In summary, we have observed coherent quench dynamics in metallic states of ultracold fermionic atoms in an optical lattice. In the hybrid Fermi–Bose system investigated here, the time evolution arises from the delocalized character of the initial fermionic state, interspecies interactions and an initial bosonic state that exhibits site-to-site fluctuations of the atom number. Such coherent dynamics also occurs in spin-1/2 interacting fermionic systems [31] , [32] and is expected to emerge in higher-spin fermionic systems [33] , following a similar quench protocol. The amplitude of the visibility oscillations depends on the single-particle correlations between the lattice sites. Therefore, coherent quench dynamics can serve as a novel tool to probe correlations in delocalized quantum phases of fermionic systems, such as the Hubbard model [34] and chains of spin-polarized fermions with intersite interactions [35] , [36] . This information is complementary to the site-resolved precision measurements of occupations in quantum gas microscopes [37] , [38] . Finally, the spectral analysis of the visibility oscillations enables precision measurements of on-site interactions and may be used to reveal complex interaction effects in hybrid quantum many-body systems. Experimental state preparation Fermi gases of 2.1(4) × 10 5 40 K atoms at a temperature of T / T F =0.20(2) and BECs of 1.7(3) × 10 5 87 Rb atoms were simultaneously created in the hyperfine states |9/2, −9/2〉 and |1, +1〉, respectively. The degenerate Fermi–Bose mixtures were held in a pancake-shaped optical dipole trap operating at λ dip =1,030 nm. The interspecies scattering length a FB between fermions and bosons was tuned by means of a Feshbach resonance, located at a magnetic field of 546.75(6) G (ref. 24 ). The 3D optical lattice ( λ lat =738 nm) was operated at blue detuning with respect to the relevant atomic transitions of both 40 K and 87 Rb. It was adiabatically ramped to a depth of for 40 K (corresponding to for 87 Rb) within 50 ms. The trapping frequencies of the horizontal and vertical confinement ( ω ⊥ , ω z ) were 2 π × (36,173) Hz for 40 K and 2 π × (25,94) Hz for 87 Rb, respectively. Then, a non-adiabatic jump into a deep lattice, for 40 K (corresponding to for 87 Rb), was performed within 50 μs, slow enough to avoid population of higher lattice bands, but fast with respect to tunnelling in the first band. Simultaneously with the lattice jump, the harmonic confinement in the horizontal plane was reduced to −2 π × 16 Hz for 40 K and 2 π × 0 Hz for 87 Rb, enhancing the coherence time of the quench dynamics [8] . In the deep lattice, the tunnelling matrix elements for fermions and bosons are J F =2 π × 33 Hz and J B =2 π × 3 Hz, respectively. The corresponding tunnelling time scales are τ F = h /( zJ F )=5.1 ms and τ B = h /( zJ B )=56 ms, where z =6 is the coordination number of a 3D lattice. For the above loading parameters, the fermions form a metallic state with trap-averaged filling per lattice site of about for vanishing Fermi–Bose interactions ( a FB ∼ 0) and about for attractive Fermi–Bose interactions ( a FB ∼ −125 a 0 ) [21] . Accordingly, the fermionic momentum distributions recorded after 9 ms time-of-flight expansion display a partially filled first Brillouin zone (see Fig. 2 ). The bosons form a BEC with a trap-averaged filling per lattice site of about and a maximal filling in the trap centre of 2.5 atoms. In-trap arrangement of atomic clouds For the above loading parameters, the horizontal and vertical in-situ Thomas–Fermi radii ( r ⊥ , r z ) are about 50 and 11 μm for 40 K and 21 and 5 μm for 87 Rb. While the total atom numbers are comparable, the fermionic cloud is about 10 times larger in volume than the bosonic one, as a consequence of Pauli pressure. The differential gravitational sag between the clouds has been measured to be 8(2) μm, leading to a notable displacement (see Supplementary Fig. 1 and Supplementary Note 1 ). Only the overlap volume of fermions and bosons (plus a thin shell of few lattice sites, which represents the coherence length of the fermions) contributes to the fermionic quench dynamics; about 5% of the fermions overlap with the bosons. This is compatible with the amplitude of the fermionic quench dynamics shown in Fig. 2c , corresponding to about 5% of the atomic density in momentum space. Spectral analysis The visibility time traces of the quench dynamics typically cover an observation time of 6 ms, sampled in steps of 40 μs. To obtain high-resolution, low-noise spectra, the time traces are processed as follows: the raw data points are interpolated using cubic splines and the origin of the time axis, t =0, corresponds to the beginning of the jump from V L to V H . To avoid distortion of the spectral analysis due to dynamics that slowly starts during the jump, the first 40 μs of the interpolated trace are removed. For times longer than the observation time, we smoothly attach an exponential decay with a time scale of about 2 ms to the interpolated curve. The such prepared curve is concatenated to its mirror image, which is obtained upon exchanging time t by − t . The resulting trace is again sampled in steps of 40 μs, and numerical Fourier analysis is performed. This processing scheme improves the data quality in two ways: First, the knowledge of the initial phase allows mirroring of the data. This doubles the size of the data set and yields a twofold improvement of the spectral resolution to about 85 Hz. Second, the additional extension of the data set by a smooth exponential decay avoids high frequency artefacts, which would arise from Fourier transform of sharp cutoffs, and makes the Fourier spectra quasi-continuous. Outline of the calculation We outline the derivation of equation (1) and discuss its extension to 3D. The Hamiltonian governing the time evolution after the quench is given by where and being bosonic and fermionic creation operators, respectively, and M is the number of lattice sites. The explicit action of the time evolution operator on the initial state is (setting ℏ =1 for convenience) We first evaluate the expectation value of the density matrix as a step towards calculating the momentum distribution, The cases m ≠ n and m = n have to be treated separately, yielding The sum in the brackets in equation (5) cannot be calculated analytically in 3D. This is due to the constraint that the fermions fill up the lowest energy states governed by E k < E F with E k =− J [cos( k x a )+cos( k y a )+cos( k z a )], where J is the hopping. In one dimension, however, the sum is easily carried out. For unconfined bosons, the site occupation | α m | 2 ≡| α | 2 is a constant equal to the mean number of bosons per site. We compute the Fourier transform of equation (5) to get the momentum distribution and integrate to obtain the visibility. This gives the expression in equation (1) for the 1D visibility. In 3D, it is possible to obtain an analytical expression for small fermionic filling, where the Fermi surface is approximately a sphere. The visibility in this case is, for k 0 < k F . Effects of harmonic confinement We assume that the single-particle ground state of a harmonically trapped system in a lattice can be described by the ground state in the continuum with a lattice renormalized mass [39] . It is not possible to analytically study a trapped lattice system. We further assume that all the bosons are in the ground state. The average on-site occupancies then take the form , where | α | 2 denotes the average occupation in the centre of the trap and is the length scale of the trap. For this case, the visibility (in the limit of low fermionic filling) is given by where and L is the length of the fermionic system. As the coordinates are rescaled, the integration is carried out over a cube of length one centred at the origin. The amplitude of oscillations in equation (7) is governed by . As | α | 2 increases, the amplitude increases for fixed . As increases with α fixed, the bosonic wave function becomes sharply peaked in space, decreasing the overlap between the bosons and the fermions. This in turn decreases the oscillation amplitude. Confinement of the bosons is therefore one reason for the reduced amplitude of oscillations seen in the experimental data. If we further include a confining trap for the fermions, one can no longer use the plane waves for the initial state. Instead, one must use fermionic harmonic oscillator states. As for the trapped bosons, we carry out calculations in the continuum as the eigenstates of harmonically trapped fermions in a lattice are not known analytically [39] , [40] . The masses of the atoms are renormalized masses obtained from the low-density limit in the lattice [39] , [40] . We get the following expression for the fermionic visibility: where are harmonic oscillator wave functions. The sum over l is shorthand for the sum over the set of quantum numbers describing a harmonic oscillator as we fill states. In the thermodynamic limit, as N →∞, the primary contribution to the first term in equation (8) comes from the diagonal part z = z ′. In this limit, the integrand is proportional to δ ( z − z ′), but the prefactor has to be determined numerically. With this, we get the compact expression where ρ F is the density of harmonically trapped fermions, given by the Thomas–Fermi formula in the thermodynamic limit. ν B,F are the inverse square length scales of the bosonic and fermionic traps, respectively. is calculated numerically from at t =0. The above expression assumes the thermodynamic limit. We have verified that calculations with experimental parameters exhibit negligible finite size effects, and the results agree with equation (9). The non-uniform spatial distribution of fermions contributes to a decrease in the oscillation amplitude. Differing confinement scales for the fermions and bosons affect the spatial overlap between them and additionally reduce the oscillation amplitude. Damping of the oscillations in the experiment is dominantly due to residual tunnelling in the post-quench system [31] and interactions between fermions and bosons in the initial state. To emphasize a key point, in all the cases we have considered, the basic time dependence of the visibility oscillations remains the same. Substructure of spectral features The comb-like substructure of the peaks in Fig. 3b originates from occupation-dependent interaction strengths , corresponding to the interaction energy of a fermion and a boson on sites that contain one fermion and n bosons [21] . Combining this modification with equations 5 and 6, the single-particle density matrix contains terms proportional to , where is independent of time. Consequently, the spectrum contains the frequencies for all integer values of n i and n j , that is, spectral features are expected at 0, How to cite this article : Will, S. et al . Observation of coherent quench dynamics in a metallic many-body state of fermionic atoms. Nat. Commun. 6:6009 doi: 10.1038/ncomms7009 (2015).